Involvement of urinary bladder Connexin43 and the circadian clock in coordination of diurnal micturition rhythm Nocturnal enuresis in children and nocturia in the elderly are two highly prevalent clinical conditions characterized by a mismatch between urine production rate in the kidneys and storage in the urinary bladder during the sleep phase. Here we demonstrate, using a novel method for automated recording of mouse micturition, that connexin43, a bladder gap junction protein, is a negative regulator of functional bladder capacity. Bladder connexin43 levels and functional capacity show circadian oscillations in wild-type mice, but such rhythms are completely lost in Cry -null mice having a dysfunctional biological clock. Bladder muscle cells have an internal clock, and show oscillations of connexin43 and gap junction function. A clock regulator, Rev-erbα, upregulates connexin43 transcription as a cofactor of Sp1, using Sp1 cis -elements of the promoter. Therefore, circadian oscillation of connexin43 is associated with the biological clock and contributes to diurnal changes in bladder capacity, which avoids disturbance of sleep by micturition. Nocturnal enuresis is the involuntary loss of urine during sleep in childhood, and nocturia is the undesired waking at night for micturition later in life. Studies show that at least 10% of school children have nocturnal enuresis [1] , [2] , and 60–90% of the elderly, over 60 years, suffer from nocturia [3] , [4] . These conditions are detrimental to the quality of life by interfering with patients' self-esteem or sleeping habits, and they are the major diseases found in urology clinics. Nocturnal enuresis and nocturia are characterized by a mismatch between urine production rate in the kidneys, and storage in the urinary bladder [5] , [6] . During the sound sleep of a healthy person, a smaller volume of urine is produced than that during the daytime, and more urine is stored during the sleep phase than during the active phase [7] , [8] , [9] . Although it is unknown how such temporal variation is generated, these phenomena could be related to biological rhythms, because behaviour, physiology and metabolism in mammals are subject to a well-controlled daily rhythm, generated by an internal self-sustained molecular oscillator referred to as the circadian clock [10] , [11] , [12] , [13] . Circadian oscillations are driven by a transcription–translation feedback loop consisting of PER and CRY as negative components and CLOCK and BMAL1 as positive components. Rhythmic oscillations of this core loop are followed by the clock-associated oscillations of Dbp and Rev-erb α, whose products regulate oscillations of a number of clock-controlled genes regulating cell- or organ-specific physiology through D-box and RORE sites, respectively [14] , [15] , [16] . These molecular oscillators exist in most body cells and organs [13] , but little is known about the role of the clock in urinary bladder function. Micturition occurs by the contraction of smooth muscles of the urinary bladder on a sensation of fullness, which is precisely controlled by regulation of the central and peripheral nerves [17] , [18] . We and others have reported that an increase in connexin43 (Cx43), a gap junction protein in the urinary bladder, enhances intercellular electrical and chemical transmission and sensitizes the response of bladder muscles to cholinergic neural stimuli. This results in a decrease in functional bladder capacity and an increase in micturition frequency in rats [19] , [20] , [21] , [22] . These phenomena mimic some aspects of an overactive bladder, a human pathological condition characterized by urinary urgency and increased micturition frequency [23] ; however, the involvement of Cx43 in regulating normal bladder function remains unclear. To further elucidate the role of Cx43 in bladder function, we investigated the effect of genetic ablation of Cx43 on micturition behaviour in mice and the implication of Cx43 for circadian micturition rhythm. The circadian micturition rhythm in free-moving mice still remains elusive, as the urine volume voided per micturition (UVVM) in mice is so minute (sometimes <50 μl) [24] , [25] . To overcome this problem, we designed a novel system, called the automated voided stain on paper (aVSOP) method, which can accurately record micturition of mice for several days. Using this system, we demonstrated the role of Cx43 and the circadian clock as regulators of functional bladder capacity in mice. We also showed that bladder muscle has internal rhythms of the clock and Cx43, which are correlated with oscillation in gap junction function. Further, we propose a novel paradigm that links the circadian clock with Cx43, in which Rev-erbα protein transactivates the Cx43 promoter through interaction with Sp1. Cx43 is involved in control of functional bladder capacity We began our study by developing an automated machine called aVSOP ( Fig. 1a ). The conversion of UVVM by mice from a drop area on filter paper has been reported to be an accurate method [24] , [26] , and this principle was applied to the automated system by using a laminated filter paper pre-treated to turn the edge of urine stains deep purple ( Supplementary Fig. S1a ). This modification enabled us to record the micturition of free-moving mice fed ad libitum for several successive days, for a UVVM as little as 10 μl ( Supplementary Fig. S1b ). 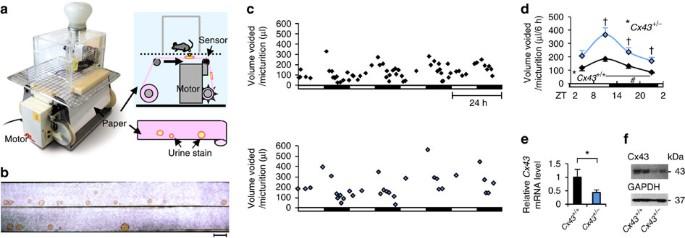Figure 1: aVSOP reveals an association between functional bladder capacity andCx43. (a) A photograph and diagram showing the aVSOP method. Each stain was traced, scanned and quantified by Image J 1.42 software. (b–d) FemaleCx43+/−mice had larger functional bladder capacity than sex-matchedCx43+/+littermates. (b) A photograph of urine spots on paper made byCx43+/+(top) andCx43+/−(bottom) mice. The scale bar indicates 10 cm, corresponding to 1 h. (c) Representative charts of UVVM ofCx43+/+(top) andCx43+/−(bottom) mice under LD conditions for 4 days. (d) UVVM per 6 h inCx43+/+andCx43+/−mice had diurnal variation (F(3[degrees of freedom (DF) for the time factor],9[error DF])=12.3 and 10.9, respectively; *P<0.005 by one-way repeated measures ANOVA;P<0.05 in the late light (sleep) phase versus late dark (active) phase, followed by Bonferroni'spost hoctest). Maximal correlations from a cosine curve (MaxCorr) ofCx43+/+andCx43+/−mice were 0.949 and 0.989, respectively: light-on at ZT0 and off at ZT12. UVVM was significantly different betweenCx43+/+andCx43+/−mice (F(1[DF for the strain factor],6[error DF])=11.2,P<0.05 by two-way repeated measures ANOVA; †P<0.05 versusCx43+/+by Bonferroni'spost hoctest;n=4 for each group, with a total of 296 micturitions). Error bars represent s.e.m. (e) RelativeCx43mRNA levels of the urinary bladder inCx43+/−andCx43+/+mice used in the micturition analysis by real-time RT–PCR. Error bars represent s.d.,n=4 for each mice. The value ofCx43+/+was set as 1. *P<0.05 by Student'st-test. (f) Cx43 protein expression of the urinary bladder inCx43+/+andCx43+/−mice. Figure 1: aVSOP reveals an association between functional bladder capacity and Cx43 . ( a ) A photograph and diagram showing the aVSOP method. Each stain was traced, scanned and quantified by Image J 1.42 software. ( b – d ) Female Cx43 +/− mice had larger functional bladder capacity than sex-matched Cx43 +/+ littermates. ( b ) A photograph of urine spots on paper made by Cx43 +/+ (top) and Cx43 +/− (bottom) mice. The scale bar indicates 10 cm, corresponding to 1 h. ( c ) Representative charts of UVVM of Cx43 +/+ (top) and Cx43 +/− (bottom) mice under LD conditions for 4 days. ( d ) UVVM per 6 h in Cx43 +/+ and Cx43 +/− mice had diurnal variation (F(3[degrees of freedom (DF) for the time factor],9[error DF])=12.3 and 10.9, respectively; * P <0.005 by one-way repeated measures ANOVA; P <0.05 in the late light (sleep) phase versus late dark (active) phase, followed by Bonferroni's post hoc test). Maximal correlations from a cosine curve (MaxCorr) of Cx43 +/+ and Cx43 +/− mice were 0.949 and 0.989, respectively: light-on at ZT0 and off at ZT12. UVVM was significantly different between Cx43 +/+ and Cx43 +/− mice (F(1[DF for the strain factor],6[error DF])=11.2, P <0.05 by two-way repeated measures ANOVA; † P <0.05 versus Cx43 +/+ by Bonferroni's post hoc test; n =4 for each group, with a total of 296 micturitions). Error bars represent s.e.m. ( e ) Relative Cx43 mRNA levels of the urinary bladder in Cx43 +/− and Cx43 +/+ mice used in the micturition analysis by real-time RT–PCR. Error bars represent s.d., n =4 for each mice. The value of Cx43 +/+ was set as 1. * P <0.05 by Student's t -test. ( f ) Cx43 protein expression of the urinary bladder in Cx43 +/+ and Cx43 +/− mice. Full size image To assess the effect of genetic Cx43 ablation on micturition, we compared heterozygous Cx43 +/− and wild-type (WT) Cx43 +/+ littermate mice by the aVSOP method ( Fig. 1b–d ), because homozygous Cx43 −/− mice die shortly after delivery [27] . Cx43 messenger RNA and protein levels in the urinary bladder of Cx43 +/− mice were decreased compared with those in Cx43 +/+ mice ( Fig. 1e,f ). In both genotypes, UVVM showed temporal variation under 12-hour light and 12-hour dark (LD) conditions ( Fig. 1b–d ), consistent with the nocturnal characteristics of the mice [28] . UVVM was higher in Cx43 +/− mice than that in Cx43 +/+ mice ( Fig. 1b–d ), while total urine volume was not significantly different ( Supplementary Fig. S1c ). These data demonstrate that the expression level of Cx43 is crucial for determining the functional capacity of the urinary bladder. This finding and the temporal variation in the micturition behaviour of the mice led us to focus on its association with Cx43 expression in the bladder and the circadian clock. Association of bladder clock with bladder capacity and Cx43 It has been reported that micturition shows a diurnal change in rodents as well as in humans [8] , [22] , [28] , [29] , although the day–night change is inverted because of the difference in diurnal versus nocturnal habits. However, it is unknown whether these changes are induced by an endogenous oscillator or only by a reflection of external LD changes. To address this in mice, we first examined micturition of WT mice under both LD and constant dark (DD) conditions. A distinct rhythm of UVVM was recorded, peaking at zeitgeber time (ZT) or circadian time (CT) 8–12 ( Fig. 2a,b ). χ 2 analysis showed a circadian periodicity under both LD and DD conditions ( Supplementary Fig. S2a ). No significant difference between LD and DD was found in the circadian amplitude (0.042 cycles per hour) quantified as relative power calculated by Fourier transform [30] ( Supplementary Fig. S2b ). This demonstrates that the mouse could be a model animal for micturition rhythmicity, and that the rhythm could be related to an internal biological rhythm that is also operational in the absence of environmental change in LD cycles. The involvement of the circadian clock in micturition behaviour was tested in mice with a dysfunctional circadian clock by deletion of Cryptochrome-1 ( Cry1 ) and Cryptochrome-2 ( Cry2 ) ( Cry -null mice); accordingly, these mice have completely arrhythmic behaviour and metabolism [11] , [31] . We placed our aVSOP system in a box with an infrared activity sensor and measured the micturition and locomotor activity, simultaneously. Similar to behavioural locomotor rhythms ( Supplementary Fig. S3a ), circadian characteristics of UVVM observed in WT mice were abolished in Cry- null mice ( Fig. 2c,d ) analysed by χ 2 and Fourier transform ( Supplementary Fig. S3b ), as well as those of total urine volume and frequency ( Supplementary Fig. S3c,d ). These findings further support the notion that the circadian clock regulates UVVM. 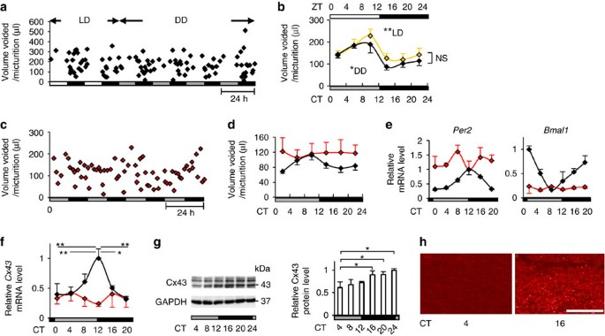Figure 2: Rhythmicity of micturition, clock genes andCx43expression in WT mice is disturbed inCry-null mice. (a) A representative chart of UVVM of WT C57BL/6 mice under LD conditions followed by DD conditions. (b) Temporal UVVM every 4 h in WT mice (n=5), for 8 days under LD conditions (940 micturitions) and 5 days under DD conditions (556 micturitions). Diurnal variation of UVVM in LD conditions (F(5,20)=17.28, **P<0.005 by one-way repeated measures ANOVA) was also observed in DD conditions (F(5,20)=8.23, *P<0.05), with no significant difference among times in LD versus DD by two-way repeated measures ANOVA. (c,d) Loss of circadian rhythm of UVVM inCry-null mice under DD conditions. Age-matched female WT, 1,493 micturitions;Cry-null, 1,009 micturitions,n=5 each. (c) A representative chart of UVVM ofCry-null mice. (d) Temporal UVVM every 4 h inCry-null (red-diamond) and WT (black-diamond) mice. Diurnal variation detected in WT mice (F(5,20)=8.21,P<0.05 by one-way repeated measures ANOVA) was not observed inCry-null mice. (e) TemporalPer2,Bmal1and (f)Cx43mRNA accumulation in the bladder in WT andCry-null mice (n=3 for each time point). MaxCorrs ofPer2,Bmal1andCx43were (0.96, 0.93 and 0.85) in WT and (0.19, 0.42 and 0.38) inCry-null mice, respectively. There was no significant difference in temporalCx43mRNA levels inCry-null mice by one-way ANOVA. (g) Immunoblots showing temporal changes in protein levels of Cx43 in WT-mouse bladder (three independent samples for each time point). (h) Immunostaining of the muscle layer in mouse urinary bladder showing a difference in immunoreactivity with a decrease in Cx43 at CT4 compared with CT16. Representative photographs of three replicated experiments with similar results are shown. Bar, 50 μm. *P<0.05 and **P<0.01 by one-way ANOVA with Tukey'spost hoctest infandg. Error bars represent s.e.m. inbandd, and s.d. ine–g. For the relative levels, the maximal values of WT were set as 1 ineandf. F(x,y),x=DF for the time factor;y=error DF inbandc. Figure 2: Rhythmicity of micturition, clock genes and Cx43 expression in WT mice is disturbed in Cry -null mice. ( a ) A representative chart of UVVM of WT C57BL/6 mice under LD conditions followed by DD conditions. ( b ) Temporal UVVM every 4 h in WT mice ( n =5), for 8 days under LD conditions (940 micturitions) and 5 days under DD conditions (556 micturitions). Diurnal variation of UVVM in LD conditions (F(5,20)=17.28, ** P <0.005 by one-way repeated measures ANOVA) was also observed in DD conditions (F(5,20)=8.23, * P <0.05), with no significant difference among times in LD versus DD by two-way repeated measures ANOVA. ( c , d ) Loss of circadian rhythm of UVVM in Cry -null mice under DD conditions. Age-matched female WT, 1,493 micturitions; Cry -null, 1,009 micturitions, n =5 each. ( c ) A representative chart of UVVM of Cry -null mice. ( d ) Temporal UVVM every 4 h in Cry -null (red-diamond) and WT (black-diamond) mice. Diurnal variation detected in WT mice (F(5,20)=8.21, P <0.05 by one-way repeated measures ANOVA) was not observed in Cry -null mice. ( e ) Temporal Per2 , Bmal1 and ( f ) Cx43 mRNA accumulation in the bladder in WT and Cry -null mice ( n =3 for each time point). MaxCorrs of Per2 , Bmal1 and Cx43 were (0.96, 0.93 and 0.85) in WT and (0.19, 0.42 and 0.38) in Cry -null mice, respectively. There was no significant difference in temporal Cx43 mRNA levels in Cry -null mice by one-way ANOVA. ( g ) Immunoblots showing temporal changes in protein levels of Cx43 in WT-mouse bladder (three independent samples for each time point). ( h ) Immunostaining of the muscle layer in mouse urinary bladder showing a difference in immunoreactivity with a decrease in Cx43 at CT4 compared with CT16. Representative photographs of three replicated experiments with similar results are shown. Bar, 50 μm. * P <0.05 and ** P <0.01 by one-way ANOVA with Tukey's post hoc test in f and g . Error bars represent s.e.m. in b and d , and s.d. in e – g . For the relative levels, the maximal values of WT were set as 1 in e and f . F( x , y ), x =DF for the time factor; y =error DF in b and c . Full size image We next examined whether the molecular machinery of the circadian clock is present in the urinary bladder. We found that the core oscillating machinery was present in the urinary bladder, as core clock genes including Per2 and Bmal1 ( Fig. 2e ), Per1, Cry1, Clock and Dbp ( Supplementary Fig. S4 ) showed characteristic circadian expression profiles by real-time RT–PCR of circadian sampling of the urinary bladder every 4 h (6 time points of the day) in WT mice. Dysfunction of the bladder circadian clock in Cry -null mice was demonstrated by a disturbed rhythm of Per2 and Bmal1 ( Fig. 2e ). We performed DNA microarray analysis to investigate the genes showing circadian rhythm in the urinary bladder more extensively. Besides the clock genes, there are thousands of oscillating genes in the bladder, as in other organs [32] , [33] . Notably, our target gene, Cx43 (also known as Gja1 ), was among the 184 genes with clear circadian rhythmicity (defined as greater than the max correlation of 0.85 from the cosine curve with a 1.5-fold amplitude of expression level [34] , [35] ) ( Supplementary Data 1 ). Cx43 mRNA showed a clear circadian rhythm with a peak at CT12 and a trough at CT0 by real-time RT–PCR ( Fig. 2f ). Cx43 protein levels remained low during the sleep phase (CT4–12), but, began to elevate 4 h after the peak of mRNA expression, and formed a plateau during the active phase (CT16–24) ( Fig. 2g ). Immunostaining of Cx43 in the muscle layer of the urinary bladder at CT4 and at CT16 also showed a clear difference in immunoreactivity ( Fig. 2h ). In rats, in which day–night difference of micturition behaviour has been described [22] , [29] , a similar correlation was observed between micturition rhythm ( Fig. 3a ), temporal variations of clock genes ( Per2 and Bmal1 ) and Cx43 mRNA expressions in the urinary bladder ( Fig. 3b ), Cx43 protein levels ( Fig. 3c ) and Cx43 immunoreactivity ( Fig. 3d ). 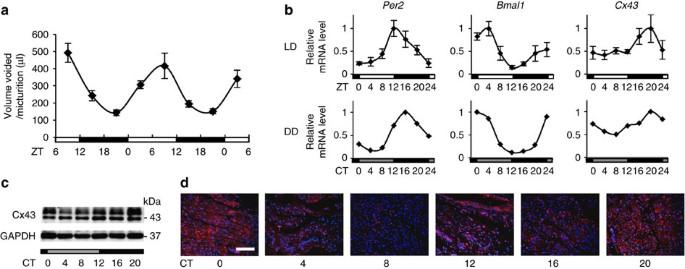Figure 3:Cx43and clock-gene expression rhythms in rats and their correlation with micturition rhythm. (a) Patterns of UVVM in female SD rats under LD conditions for 2 days (n=15, 1,001 micturitions; F(2.7[degrees of freedom [DF] for the time factor],38.3[error DF])=11.9; *P<0.005 by one-way repeated measures ANOVA with a Greenhouse–Geisser correction). (b) Temporal mRNA accumulation ofPer2 Bmal1andCx43in the rat bladder under LD and DD conditions (n=5 andn=2 for each time point, respectively). MaxCorrs were 0.87, 0.90 and 0.84 in LD conditions, respectively, and 0.98, 0.95 and 0.93 in DD conditions, respectively. (c) Temporal Cx43 protein accumulation in the rat bladder under DD conditions as shown by immunoblotting. (d) Immunostaining of Cx43 in the rat bladder under DD conditions (red, Cx43; blue, DAPI). The scale bar indicates 100 μm. Error bars represent s.e.m. ina, and s.d. inb. For the relative expression, maximal values were set as 1 inb. Figure 3: Cx43 and clock-gene expression rhythms in rats and their correlation with micturition rhythm. ( a ) Patterns of UVVM in female SD rats under LD conditions for 2 days ( n =15, 1,001 micturitions; F(2.7[degrees of freedom [DF] for the time factor],38.3[error DF])=11.9; * P <0.005 by one-way repeated measures ANOVA with a Greenhouse–Geisser correction). ( b ) Temporal mRNA accumulation of Per2 Bmal1 and Cx43 in the rat bladder under LD and DD conditions ( n =5 and n =2 for each time point, respectively). MaxCorrs were 0.87, 0.90 and 0.84 in LD conditions, respectively, and 0.98, 0.95 and 0.93 in DD conditions, respectively. ( c ) Temporal Cx43 protein accumulation in the rat bladder under DD conditions as shown by immunoblotting. ( d ) Immunostaining of Cx43 in the rat bladder under DD conditions (red, Cx43; blue, DAPI). The scale bar indicates 100 μm. Error bars represent s.e.m. in a , and s.d. in b . For the relative expression, maximal values were set as 1 in b . Full size image The circadian change of mRNA was reflected in the protein level, and the increase/decrease in Cx43 protein expression correlated with the decrease/increase of UVVM, respectively, in WT mice and rats. Similarly, Cry -null mice tended to show a constantly low level of Cx43 mRNA ( Fig. 2f ) with a high level of UVVM ( Fig. 2d ). This inverse expression can be accounted for by altered bladder sensitivity caused by a differential level of gap junction formation by Cx43, because the half-life of connexin proteins is up to 5 h and expression largely follows transcript levels [36] , [37] . These findings suggest that the bladder circadian clock coordinates UVVM via circadian regulation of Cx43 gene expression. Internal oscillations of bladder clock and Cx43 function We investigated if the circadian clock oscillates in the bladder without systemic control. Therefore, we investigated its oscillation in ex vivo bladder in culture. We used mice carrying a PER2::LUC fusion protein, which has been engineered to produce bioluminescence, when the clock gene Per2 is activated in the presence of luciferin [38] . The ex vivo slice culture of the bladder from Per2 :: luc mice demonstrated a robust oscillation of bioluminescence in the muscle layer of the bladder for at least four cycles ( Fig. 4a ; Supplementary Movie 1 ). The oscillation continued for ~2 months in the medium changed every 5 days. This oscillation was not observed in Per2 :: luc mice with the Clock -mutation ( Clk Δ 19 /Clk Δ 19 ) ( Supplementary Fig. S5 ). These findings clearly demonstrate that a functional circadian clock exists in the smooth muscle of the urinary bladder. 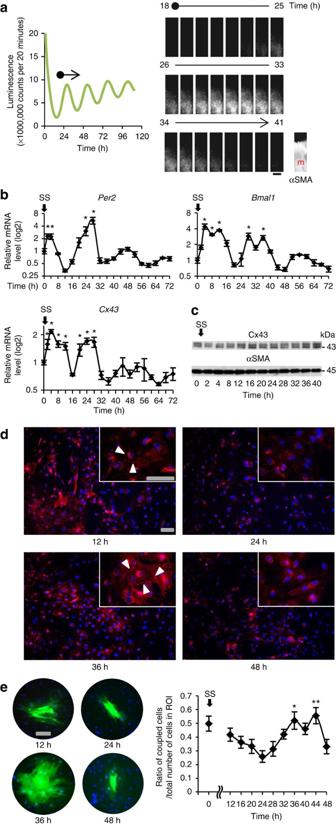Figure 4: Oscillation of the circadian clock,Cx43and gap junction function in bladder muscle cells without systemic control. (a) Oscillation of luminescence in bladderex vivoslice culture obtained from mPer2Luciferaseknock-in (Per2::luc) mice. The period of oscillation was 24.92±0.56 (mean±s.d.) (n=10). The muscle layer of the bladder is shown by alpha smooth muscle actin (αSMA) immunostaining. m, muscle. The scale bar indicates 100 μm. The oscillation of luminescence is also shown by a movie inSupplementary Movie 1. (b) Temporal variation ofPer2,Bmal1andCx43mRNA levels in serum-shocked rat BSMC. *P<0.01 against the nadir of each genes' mRNA levels (time 12 forPer2, time 48 forBmal1and time 64 forCx43) by one-way ANOVA with Dunnett'spost hoctest (n=3–6). SS, serum shock. For relative levels, the values before serum shock were set as 1. (c) Immunoblots showing temporal changes in Cx43 protein levels with αSMA as a loading control in serum-shocked rat BSMC. (d) Immunostaining of Cx43 at times 12, 24, 36 and 48 h in serum-shocked rat BSMC (red, Cx43; blue, DAPI). Arrow heads indicate typical plaques of gap junctions. Representative images of two replicate experiments with similar results are shown incandd. (e) Oscillation of gap junction function evaluated by Lucifer yellow microinjection in serum-shocked rat BSMC. One representative photograph of each time point (green, Lucifer yellow; blue, Hoechst 33342) and overall quantification of the degree of dye-coupling (n=6–9, a total of 71 injections) is shown. *P<0.05 and **P<0.01 versus time 24 h by one-way ANOVA with Tukey-Kramer'spost hoctest. Similar significant differences were obtained in two independent experiments. Error bars represent s.e.m. inbande. Scale bars indandeindicate 100 μm. Figure 4: Oscillation of the circadian clock, Cx43 and gap junction function in bladder muscle cells without systemic control. ( a ) Oscillation of luminescence in bladder ex vivo slice culture obtained from m Per2 Luciferase knock-in ( Per2 :: luc ) mice. The period of oscillation was 24.92±0.56 (mean±s.d.) ( n =10). The muscle layer of the bladder is shown by alpha smooth muscle actin (αSMA) immunostaining. m, muscle. The scale bar indicates 100 μm. The oscillation of luminescence is also shown by a movie in Supplementary Movie 1 . ( b ) Temporal variation of Per2 , Bmal1 and Cx43 mRNA levels in serum-shocked rat BSMC. * P <0.01 against the nadir of each genes' mRNA levels (time 12 for Per2 , time 48 for Bmal1 and time 64 for Cx43 ) by one-way ANOVA with Dunnett's post hoc test ( n =3 – 6). SS, serum shock. For relative levels, the values before serum shock were set as 1. ( c ) Immunoblots showing temporal changes in Cx43 protein levels with αSMA as a loading control in serum-shocked rat BSMC. ( d ) Immunostaining of Cx43 at times 12, 24, 36 and 48 h in serum-shocked rat BSMC (red, Cx43; blue, DAPI). Arrow heads indicate typical plaques of gap junctions. Representative images of two replicate experiments with similar results are shown in c and d . ( e ) Oscillation of gap junction function evaluated by Lucifer yellow microinjection in serum-shocked rat BSMC. One representative photograph of each time point (green, Lucifer yellow; blue, Hoechst 33342) and overall quantification of the degree of dye-coupling ( n =6 – 9, a total of 71 injections) is shown. * P <0.05 and ** P <0.01 versus time 24 h by one-way ANOVA with Tukey-Kramer's post hoc test. Similar significant differences were obtained in two independent experiments. Error bars represent s.e.m. in b and e . Scale bars in d and e indicate 100 μm. Full size image We then examined cultured bladder smooth muscles cells (BSMC) under serum shock, an in vitro model of genetic oscillation [39] . After serum shock in BSMC, autonomous oscillation of clock genes ( Per2 and Bmal1 ) was observed ( Fig. 4b ). Concurrently, Cx43 levels also showed autonomous rhythmicity ( Fig. 4b ), which was followed by a change in protein levels ( Fig. 4c,d ), as observed in the bladder in vivo ( Figs 2f–h and 3b–d ). This change occurred in parallel with a change in cell–cell communication rate as shown by a dye-transfer experiment with Lucifer yellow microinjected intracellularly ( Fig. 4e ). At 24 h after the initiation of rhythm when Cx43 protein levels were close to their nadir, the amount of dye-transferred cells was at its minimum. However, at 36 h when Cx43 protein levels were close to their peak, the amount of dye-transferred cells was considerably increased (more than twofold compared with the minimum level at 24 h). These findings clearly demonstrate that bladder muscle cells have an internal rhythm generating system, which elicits oscillation in gap junction function. Activation of Cx43 promoter by a clock component Rev-erbα We next investigated the molecular mechanism of Cx43 regulation by the clock. We searched for E-box, D-box and RORE sequences in the 5′ prime region of Cx43 , because clock genes are known to regulate clock-controlled genes by binding to these sequences [15] , [40] , [41] . However, we identified no such canonical sequences in a species-conserved manner within 10,000 bases from the transcription start site* (*for RORE, there are 3 atypical RORE sequences detected from −720 to −467, but their transcriptional role for Cx43 was negated as shown in Supplementary Fig. S6 and Supplementary Discussion ). Therefore, we suspected that the circadian clock might regulate the Cx43 promoter by a novel mechanism. We examined the effect of clock genes on the Cx43 promoter by promoter-reporter assays in HEK293T cells using a pGL-2-mouse Cx43- promoter–reporter construct containing −1686/+165 (ref. 42 ). There was little effect of Clock/Bmal1 and Cry1 (positive and negative regulators of genes with E-box elements as shown for the Per1 promoter) or of Dbp and E4bp4 (regulators of genes with D-box elements as shown for the Per1 promoter) on the Cx43 promoter ( Supplementary Fig. S7a,b ). A RORE-binding protein, Rorα, also did not have any effect on Cx43 promoter activity. However, Rev-erbα, which has been reported as a negative competitor of Rorα [43] (as shown for the Bmal1 promoter, Supplementary Fig. S7c ), markedly increased Cx43 promoter activity ( Supplementary Fig. S7a ) in a dose-dependent manner ( Fig. 5a ), while the application of various concentrations of a mutant Rev-erbα (Rev-erbα-truncated mutant deleted with 127–206 amino acids) failed to activate the Cx43 promoter ( Fig. 5b ). 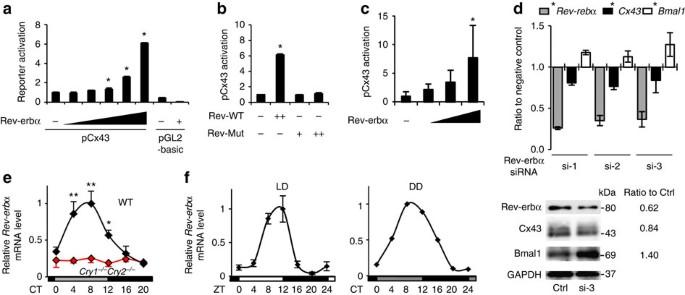Figure 5: Rev-erbα upregulates Cx43 expression. (a) Dose-dependent activation ofCx43transcription by Rev-erbα in HEK293T cells (n=3 for each dose). (b) Impaired activation ofCx43transcription by a mutant of Rev-erbα without 127–206 amino acids from the N-terminal (Rev-Mut) in HEK293T cells (n=3 for each dose). (c) Activation ofCx43transcription by Rev-erbα in rat BSMC (n=6 for each dose). *P<0.01 versus Rev-erbα (−) by one-way ANOVA with Dunnett'spost hoctest ina–c. Similar data obtained in three independent experiments foraandb, and in two independent experiments forc. (d) Suppression of Cx43 expression by knock-down of endogenous Rev-erbα in BSMC. Three types ofRev-erbα siRNAs, containing high (si-1), middle (si-2) and low (si-3) GC ratios or their controls containing corresponding GC ratios were transfected. (n=4). mRNA and protein expression (data of si-3) was normalized by 18 s ribosomal RNA and GAPDH, respectively. Interference ofRev-erbα mRNA significantly decreased mRNA expression ofCx43and increasedBmal1compared with their corresponding controls (F(1[DF for the treatment factor],18[error DF])=324 forRev-erbα, 9.7 forCx43and 11.7 forBmal1.*P<0.01 by two-way ANOVA). Temporal bladderRev-erbα mRNA accumulation in WT andCry-null mice (n=3). (e) and in rats under LD (n=5) and DD (n=2) conditions (f). *P<0.05 versus CT8 and **P<0.01 versus CT0, 16 and 20 in WT by one-way ANOVA with Tukey'spost hoctest. No significant difference inCry-null mice. MaxCorrs were WT, 0.98;Cry-null, 0.31; rats in LD, 0.84; in DD, 0.93. The maximal value of WT was set as 1. Error bars represent s.d. ina–f. For relative levels, Rev-erbα (−) was set as 1 ina–c. Figure 5: Rev-erbα upregulates Cx43 expression. ( a ) Dose-dependent activation of Cx43 transcription by Rev-erbα in HEK293T cells ( n =3 for each dose). ( b ) Impaired activation of Cx43 transcription by a mutant of Rev-erbα without 127–206 amino acids from the N-terminal (Rev-Mut) in HEK293T cells ( n =3 for each dose). ( c ) Activation of Cx43 transcription by Rev-erbα in rat BSMC ( n =6 for each dose). * P <0.01 versus Rev-erbα (−) by one-way ANOVA with Dunnett's post hoc test in a – c . Similar data obtained in three independent experiments for a and b , and in two independent experiments for c . ( d ) Suppression of Cx43 expression by knock-down of endogenous Rev-erbα in BSMC. Three types of Rev-erb α siRNAs, containing high (si-1), middle (si-2) and low (si-3) GC ratios or their controls containing corresponding GC ratios were transfected. ( n =4). mRNA and protein expression (data of si-3) was normalized by 18 s ribosomal RNA and GAPDH, respectively. Interference of Rev-erb α mRNA significantly decreased mRNA expression of Cx43 and increased Bmal1 compared with their corresponding controls (F(1[DF for the treatment factor],18[error DF])=324 for Rev-erb α, 9.7 for Cx43 and 11.7 for Bmal1. * P <0.01 by two-way ANOVA). Temporal bladder Rev-erb α mRNA accumulation in WT and Cry -null mice ( n =3). ( e ) and in rats under LD ( n =5) and DD ( n =2) conditions ( f ). * P <0.05 versus CT8 and ** P <0.01 versus CT0, 16 and 20 in WT by one-way ANOVA with Tukey's post hoc test. No significant difference in Cry -null mice. MaxCorrs were WT, 0.98; Cry -null, 0.31; rats in LD, 0.84; in DD, 0.93. The maximal value of WT was set as 1. Error bars represent s.d. in a – f . For relative levels, Rev-erbα (−) was set as 1 in a – c . Full size image Additionally, in BSMC, Rev-erbα dose-dependently upregulated Cx43 promoter activity ( Fig. 5c ). Conversely, inhibition of Rev-erbα by short interfering RNA (siRNA) decreased Cx43 mRNA and protein expression ( Fig. 5d ), while the same siRNA enhanced expression of Bmal1. These results suggest that Cx43 activation is elicited through an unreported positive transcriptional control by Rev-erbα. Rev-erb α mRNA showed a clear circadian rhythm in mouse and rat urinary bladders with a peak time at CT/ZT 4–12 and a trough at CT/ZT16–24 ( Fig. 5e,f ). In Cry -null mice, Rev-erb α mRNA stayed arrhythmic at a lower level ( Fig. 5e ). These two patterns are consistent with the role of Rev-erbα as a positive regulator for Cx43, because the Cx43 expression profile showed a peak at CT/ZT12–20 and a trough at CT/ZT0–8 in WT mice and rats, but stayed arrhythmic at a lower level in Cry -null mice ( Figs 2f and 3b ). Sp1-dependent activation of Cx43 transcription by Rev-erbα To clarify the novel molecular mechanism of Rev-erbα on promoter activity, we first attempted to identify the site with effects on the Cx43 promoter by a deletion experiment because the 5′-region of Cx43 contains several cis -elements including AP-1, AP-2, Sp1, half ERE, and cAMP-response element [44] . Truncated −700/+165, −300/+165 and −147/+165 constructs did not affect the activation of the Cx43 promoter by Rev-erbα. In contrast, the transcription activation of Cx43 by Rev-erbα was markedly diminished in the −54/+165 and −44/+165 constructs ( Fig. 6a ). 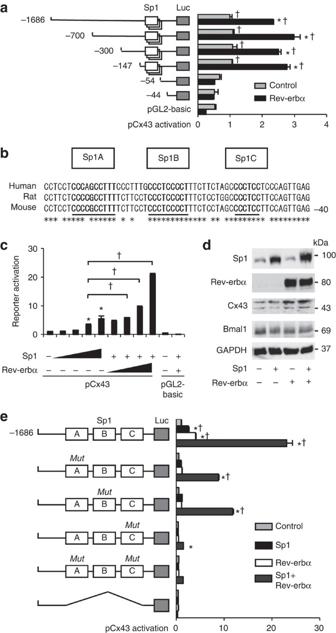Figure 6: Sp1-dependent activation of Cx43 expression by Rev-erbα. (a) Sequences including Sp1 sites are indispensable forCx43promoter activation by Rev-erbα. *P<0.001 versus the control of each construct and †P<0.001 versus −54 (without Sp1 sequences) construct by two-way ANOVA with Bonferroni'spost hoctest (n=3 for each). (b–e) Rev-erbα and Sp1 activateCx43expression using Sp1 sites. (b) Diagram ofCx43promoter sequences including three Sp1 sites, labelled as Sp1A, B and C. The asterisk indicates corresponding nucleotide sequences among humans, rats and mice. (c) Dose-dependent activation ofCx43transcription by Sp1 and Rev-erbα with Sp1. *P<0.001 versus the value -without Sp1 and Rev-erbα, and †P<0.001 by one-way ANOVA with Tukey'spost hoctest (n=3 for each). (d) Immunoblot analysis of the effect of Sp1 and Rev-erbα on expression of Cx43 and Bmal1 (control of negative regulatory effect by Rev-erbα). (e) Impaired activation of pCx43 with the Sp1 sites mutation by Sp1 and Rev-erbα. *P<0.001 versus the controls of each construct, and †P<0.001 versus theMutC construct by two-way ANOVA with Bonferroni'spost hoctest (n=3 for each group). Error bars represent s.d. ina,cande. Cells used were HEK293T in all transfection experiments. The control without Rev-erbα and Sp1 was set as 1 ina,cande. One representative of two experiments with similar results is shown ina,c,dande. Figure 6: Sp1-dependent activation of Cx43 expression by Rev-erbα. ( a ) Sequences including Sp1 sites are indispensable for Cx43 promoter activation by Rev-erbα. * P <0.001 versus the control of each construct and † P <0.001 versus −54 (without Sp1 sequences) construct by two-way ANOVA with Bonferroni's post hoc test ( n =3 for each). ( b – e ) Rev-erbα and Sp1 activate Cx43 expression using Sp1 sites. ( b ) Diagram of Cx43 promoter sequences including three Sp1 sites, labelled as Sp1A, B and C. The asterisk indicates corresponding nucleotide sequences among humans, rats and mice. ( c ) Dose-dependent activation of Cx43 transcription by Sp1 and Rev-erbα with Sp1. * P <0.001 versus the value -without Sp1 and Rev-erbα, and † P <0.001 by one-way ANOVA with Tukey's post hoc test ( n =3 for each). ( d ) Immunoblot analysis of the effect of Sp1 and Rev-erbα on expression of Cx43 and Bmal1 (control of negative regulatory effect by Rev-erbα). ( e ) Impaired activation of pCx43 with the Sp1 sites mutation by Sp1 and Rev-erbα. * P <0.001 versus the controls of each construct, and † P <0.001 versus the Mut C construct by two-way ANOVA with Bonferroni's post hoc test ( n =3 for each group). Error bars represent s.d. in a , c and e . Cells used were HEK293T in all transfection experiments. The control without Rev-erbα and Sp1 was set as 1 in a , c and e . One representative of two experiments with similar results is shown in a , c , d and e . Full size image Between −147 and −54 of the Cx43 promoter, there are cis -elements evolutionally conserved among humans, rats and mice including three putative GC-rich Sp1-binding sites ( Fig. 6b ) [45] , [46] . Exogenous expression of a transcription factor Sp1 activated the Cx43 promoter in a dose-dependent manner, and its effect was dramatically increased by the addition of exogenous Rev-erbα ( Fig. 6c ). Protein expression of Cx43 was also upregulated by exogenous Sp1 and Rev-erbα ( Fig. 6d ). The promoter activation induced by Sp1/Rev-erbα was inhibited by mutations of the three Sp1 cis -elements, in which the proximal was most crucial (Sp1C in Fig. 6e ), and was completely abolished by deletion of all Sp1 sites ( Fig. 6e ). Sp3, another activator bound to Sp1 sites of Cx43 promoter [45] , also enhanced Cx43 promoter activity in the presence of Rev-erbα ( Supplementary Fig. S8 ), supporting the involvement of Sp1 sites for enhancement of Cx43 transcription by Rev-erbα. In conclusion, unlike the negative transcriptional role of Rev-erbα using RORE sites, the novel positive transcriptional role of Rev-erbα requires Sp1 cis -elements on the Cx43 promoter. Rhythmic assembly of Rev-erbα and Sp1 at Cx43 promoter We hypothesized that Rev-erbα acts as a cofactor of Sp1, because Rev-erbα dose-dependently enhanced Cx43 activation by Sp1. To determine whether Rev-erbα interacts with Sp1 at Sp1 sites of the Cx43 promoter, a co-immunoprecipitation assay and chromatin immunoprecipitation assay (ChIP) were performed in HEK293T cells transfected with HA-Rev-erbα and DDDDK-Sp1 (protein expression of these constructs are shown in Supplementary Fig. S9 ). We observed a DDDDK-Sp1 band in immunoprecipitates with an anti-HA antibody, and HA-Rev-erbα was detected in immunoprecipitates with an anti-DDDDK antibody ( Fig. 7a ), indicating that Rev-erbα can form a complex with Sp1. The ChIP assay revealed that, in immunoprecipitates of the chromatin fragments using antibodies for HA and DDDDK, specific enrichment was obtained by primers targeted on Sp1 cis -elements of the human Cx43 promoter ( Fig. 7b ). These findings demonstrate that Rev-erbα interacts with Sp1 at Sp1 sites of the Cx43 promoter. 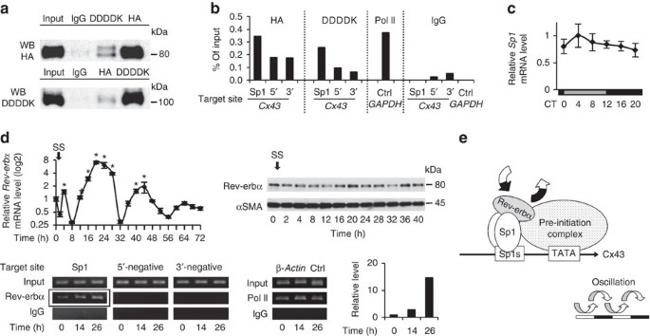Figure 7: Rhythmic assembly of Rev-erbα and Sp1 at Sp1 sites of theCx43promoter. (a) Co-immunoprecipitation showing a complex formation between HA-tagged Rev-erbα and DDDDK-tagged Sp1 transfected in HEK293T cells, using antibodies for HA and DDDDK. One representative of three experiments with similar results is shown. (b) ChIP assay using antibodies for HA and DDDDK in HEK 293T cells transfected with HA-Rev-erbα and DDDDK-Sp1. Analyses by real-time RT–PCR are shown, targeted against endogenous Sp1 sites of the humanCx43promoter and its negative control sites, which are ~7 kbp up- (5′) and 10 kbp down- (3′) stream from the transcription start site. A ChIP assay using an antibody for RNA polymerase II and primers for humanGAPDHpromoter was used as a positive control. One representative of two experiments with similar results is shown. (c) TemporalSp1mRNA accumulation in the mouse bladder (n=3 for each time point). There were no significant differences among time points by one-way ANOVA. (d) Oscillations ofRev-erbα mRNA (left) and protein expression (right) in serum-shocked rat BSMC (top row). *P<0.01 versus the nadir value (time 8) by one-way ANOVA with Dunnett'spost hoctest (n=3–6). SS, serum shock. The ChIP assay, using an antibody for endogenous Rev-erbα, was analysed by RT–PCR targeted against endogenous Sp1 sites of the ratCx43promoter and negative control sites, which are ~8 kbp up- (5′-negative) and down- (3′-negative) stream (bottom row). β-Actinis a positive control. Results of real-time RT–PCR are added; it was targeted against Sp1 sites of theCx43promoter, which was immunoprecipitated using an antibody for Rev-erbα (corresponding to the framed bands, bottom). One representative of two experiments with similar results is shown. (e) A mechanistic scheme ofCx43oscillation, controlled by the Rev-erbα and Sp1 complex binding to Sp1 sites of theCx43promoter. Error bars represent s.d. inc, and s.e.m. ind. For relative levels, the maximal value was set as 1 inc, and the values before serum shock (time 0) was set as 1 ind. Figure 7: Rhythmic assembly of Rev-erbα and Sp1 at Sp1 sites of the Cx43 promoter. ( a ) Co-immunoprecipitation showing a complex formation between HA-tagged Rev-erbα and DDDDK-tagged Sp1 transfected in HEK293T cells, using antibodies for HA and DDDDK. One representative of three experiments with similar results is shown. ( b ) ChIP assay using antibodies for HA and DDDDK in HEK 293T cells transfected with HA-Rev-erbα and DDDDK-Sp1. Analyses by real-time RT–PCR are shown, targeted against endogenous Sp1 sites of the human Cx43 promoter and its negative control sites, which are ~7 kbp up- (5′) and 10 kbp down- (3′) stream from the transcription start site. A ChIP assay using an antibody for RNA polymerase II and primers for human GAPDH promoter was used as a positive control. One representative of two experiments with similar results is shown. ( c ) Temporal Sp1 mRNA accumulation in the mouse bladder ( n =3 for each time point). There were no significant differences among time points by one-way ANOVA. ( d ) Oscillations of Rev-erb α mRNA (left) and protein expression (right) in serum-shocked rat BSMC (top row). * P <0.01 versus the nadir value (time 8) by one-way ANOVA with Dunnett's post hoc test ( n =3 – 6). SS, serum shock. The ChIP assay, using an antibody for endogenous Rev-erbα, was analysed by RT–PCR targeted against endogenous Sp1 sites of the rat Cx43 promoter and negative control sites, which are ~8 kbp up- (5′-negative) and down- (3′-negative) stream (bottom row). β -Actin is a positive control. Results of real-time RT–PCR are added; it was targeted against Sp1 sites of the Cx43 promoter, which was immunoprecipitated using an antibody for Rev-erbα (corresponding to the framed bands, bottom). One representative of two experiments with similar results is shown. ( e ) A mechanistic scheme of Cx43 oscillation, controlled by the Rev-erbα and Sp1 complex binding to Sp1 sites of the Cx43 promoter. Error bars represent s.d. in c , and s.e.m. in d . For relative levels, the maximal value was set as 1 in c , and the values before serum shock (time 0) was set as 1 in d . Full size image We next examined whether the endogenous Rev-erbα/Sp1 complex is rhythmically formed on Sp1 sites of the Cx43 promoter. It is likely that Rev-erbα, but not Sp1, could contribute to the rhythmic formation of the Rev-erbα/Sp1 complex, because Sp1 mRNA showed no marked rhythm ( Fig. 7c ), in contrast with the strong rhythm of Rev-erb α mRNA in the bladder ( Fig. 5e,f ). To verify the rhythmic role of Rev-erbα estimated in vivo , we applied rat BSMC under serum shock in vitro for the ChIP assay on the Cx43 promoter using an anti-Rev-erbα antibody. After confirming the circadian expression of Rev-erb α mRNA and protein ( Fig. 7d ), we collected the cells before serum shock, and 14 h and 26 h after serum shock. At 26 h the level of Rev-erbα detected on Sp1 sites of the Cx43 promoter was higher than that at 14 h ( Fig. 7d ), when Cx43 mRNA expression showed a peak and nadir, respectively ( Fig. 4b ). Therefore, we conclude that this rhythmic formation of the Rev-erbα/Sp1 complex on the Sp1 sites of Cx43 promoter is one mechanism that the clock induces for circadian oscillation of Cx43 expression ( Fig. 7e ). Day-night micturition rhythm in humans enables a sound sleep during the sleep phase. This rhythm is not simply caused by a higher water intake during the day, because temporal variation in urine production is maintained in subjects under constant routine, when food and drink are taken equally during 24 h (ref. 47 ). In physiological conditions, nocturnal micturition is prevented not only by a decrease in urine production rate from the kidneys, but also by an increase in storage capacity of the urinary bladder [7] , [8] , [9] . Day–night differences in bladder capacity are experienced in the daily life of humans and their disturbance can be seen in disorders such as nocturnal enuresis and nocturia. The treatment of these patients in clinics is often limited to palliation because the precise mechanism underlying the micturition rhythm is unknown. In the beginning of the current study, we aimed to use a mouse model with/without genetic modification for investigating this mechanism. A day-night difference in micturition is known to exist in humans and rodents [8] , [22] , [28] , [29] , but circadian analysis of micturition in mice has been precluded by the difficulty in diachronic measuring of urine volume with high accuracy. To overcome these problems, we designed the aVSOP system, which enabled an accurate record of minute micturition volume as little as 10 μl for several days. This method clearly recorded circadian rhythm of micturition in mice (also avoiding micturition during the sleep phase), suggesting that this rhythm should have a mechanism conserved among species. The aVSOP method also enabled us to use genetically engineered mice for unravelling the molecular events responsible for controlling micturition. In Cx43 +/− mice, this method showed the importance of Cx43 for determining functional bladder capacity, and in Cry -null mice, it showed a novel function of the circadian clock: circadian regulation of functional bladder capacity. Oscillation of the internal clock was demonstrated in the urinary bladder muscle layer ex vivo and in cultured BSMC, in parallel with the functional change in gap junctions, compatible with the rhythm of Cx43 levels. Collectively, these findings constitute the key concept of this study: the clock elicits oscillation in Cx43 levels and sensitivity of BSMC, which contribute to altered functional bladder capacity and micturition frequency during the 24-h cycle. Micturition during the sleep phase is undesirable for humans, in terms of arousal from sleep, hygiene or maintenance of body temperature, which could also be applicable to rodents. By focussing on Cx43 in the urinary bladder and the circadian clock in the present study, we showed a novel aspect in normal and pathological physiology of the diurnal micturition rhythm. However, we should also note that Cx43 in the bladder is not the only determinant of this rhythm. Enuresis and nocturia are caused not only by decreased functional bladder capacity, but also by impairment of cortical arousal level in the brain, urine production rhythm in the kidneys [4] , and the interaction between each other [48] . In the bladder, there are also many other candidate molecules with diurnal oscillation, as listed in our microarray data ( Supplementary Data 1 ), such as genes associated with smooth muscle contraction ( Cacna1g, Ednrb and Gucy1a3 ) or response to pain ( Slc6a2, Ednrb and Grik1 ). These genes could also be contributing to micturition rhythm. Future studies may elucidate the association of these factors with the circadian clock, and the aVSOP method could serve as an important tool for that purpose. The molecular mechanism of Cx43 oscillation that may underlie these phenomena is also noteworthy. Rev-erbα protein, known as a constitutive repressor [43] , [49] , acts as a transcriptional activator for Cx43 by luciferase-reporter assay. Intriguingly, for Cx43 activation, Rev-erbα does not require a canonical RORE site, but acts indirectly on Sp1 sites by interacting with Sp1 protein. This is similar to previous reports showing the physical interaction of Sp1 and nuclear receptors, such as RAR, RXR, ERs and PPARγ [50] , [51] , [52] . The identification of a co-activator-like function of Rev-erbα advocates a novel paradigm for controlling circadian gene expression: circadian clock components can modulate the activity of transcription factors coded by non-clock genes by functioning as transcriptional cofactors. Genome-wide screening of putative clock-associated sequences has revealed that many genes showing circadian oscillation do not have binding sequences for clock proteins [14] , [15] , and our finding suggests that these genes could possibly be regulated by clock proteins acting as cofactors. In summary, the circadian clock is associated with the oscillating expression of Cx43 in BSMC via a previously unknown regulatory mechanism, and it contributes to changes in bladder capacity with an increase during the sleep phase and a decrease during the active phase. This study warrants chronobiological approaches for the investigation and treatment of nocturnal enuresis and nocturia. Animals Female Cx43 heterozygote KO mice ( Cx43 +/− ) [53] aged 16–21 weeks, their female WT littermates ( Cx43 +/+ ), and female Cry1 −/− Cry2 −/− mice ( Cry -null) [11] aged 10 weeks were used. C57BL/6 mice and Sprague Dawley (SD) female rats were purchased from Japan Lab Animals and Japan SLC. Animals were treated in accordance with NIH animal care guidelines, and the Kyoto University Animal Experiment Committee approved all animal experiments. Micturition analysis in mice Micturition assessment machines for aVSOP were manufactured by Real-designs(Kyoto, Japan). Rolled laminated filter paper, pre-treated to turn the edge of urine stains deep purple, was wound up at a speed of 10 cm per hour under a water-repellent wire lattice. Urine stains were counted and traced to convert micturition volume by the formula of a standard curve, calculated by the correlation of normal saline and the stained area ranging from 10–800 μl. Cx43 +/− and Cx43 +/+ mice were kept in a cage with the dimensions of 110 mm×160 mm×75 mm (height×depth×width), measured under LD conditions for 4 days and killed for RNA extraction. The male WT mice were measured for 8 days under LD and followed by 5 days under DD conditions. The female WT and Cry -null mice were kept in a cage with dimensions of 75 mm×160 mm×75 mm, and measured with a simultaneous actogram under DD conditions, for 5 days. Total urine volume per hour was estimated by dividing the volume by the time interval between the given and preceding voiding (filling time), when the filling time was more than 1 h (ref. 7 ). Micturition analysis in rats Micturition of SD rats was recorded by an electronic balance system [22] under LD conditions for 2 days. Real-time RT–PCR analysis Female C57BL/6 mice aged 8 weeks and Cry -null mice aged 10 weeks were killed every 4 h at 6 time points during the day under a dim light ( n =3 for each time per strain) after acclimation for 2 weeks, under LD conditions followed by DD conditions. Female SD rats aged 7 weeks were acclimated for a week under LD conditions and killed at every 4 h ( n =5 for each time), followed by DD conditions, and then killed in the same manner ( n =2 for each time). Complementary DNA was synthesized from 1 μg of RNA extracted from the bladder and cultured cells, using a Superscript VILO cDNA Synthesis Kit (Invitrogen). Primers used are listed in Supplementary Table S1 . Real-time RT–PCR was performed using SYBR Green PCR Master Mix with 7500 Fast Real-Time PCR system (Applied Biosystems) [22] . Each sample was normalized against an internal 18 s ribosomal RNA control (Takara). Maximal correlation coefficients (MaxCorr) were calculated using Mathematica ver. 5.1 according to a modified program [35] . Immunoblotting Whole-cell lysates from bladder tissues and cultured cells were lysed with radioimmunoprecipitation assay buffer containing proteinase inhibitors, which were resolved by SDS–PAGE and transferred to an Immobilon-P membrane. The membranes were incubated with antibodies against Cx43 (Zymed, 1:200; Sigma-Aldrich, 1:1000), Rev-erbα (Cell Signaling Technology, 1:500; Abcam, 1:600), Bmal1 (Santa Cruz, 1:200), Sp1 (Millipore, 1:2000), αSMA (Sigma-Aldrich, 1:5000), Sp3 (BioLegend, 1:500), HA (Abcam, 1:8000), DDDDK (MBL, 1:2000) and GAPDH (Cell Signaling, 1:2000). The immunoreactivities were visualized with enhanced chemiluminescence using HRP-conjugated anti-rabbit or mouse IgG antibody (Pierce) [22] . Bioluminescence recording Slice cultures of bladder were obtained from adult Period2 Luciferase knock-in ( Per2luc ) mice [38] (Jackson Laboratories), and Per2 :: luc mice with a Clock mutation ( Clk Δ 19 /Clk Δ 19 ) generated by crossing Per2 :: luc mice to Clock mutant (Clk Δ19 /Clk Δ19 ) mice (Jackson Laboratories). The slice cultures were kept at 36 °C with culture medium containing 1 mM luciferin [54] . Bioluminescence was measured with a highly sensitive cryogenic CCD camera (Spectra Video SV16KV/CT: PixelVision) equipped with a microscope (Carl Zeiss) [55] . Immunostaining of the urinary bladder Mice bladder tissues and slice cultures were fixed with 4% paraformaldehyde in 0.1 M. phosphate buffer (0.1MPB, pH 7.4) for 24 h (ref. 54 ). After embedding bladder tissues in paraffin, we cut 5-μ thick sections with a microtome. After being treated with 1% BSA, sections were incubated with Cx43 rabbit polyclonal antibody (Invitrogen, 1:50) or αSMA (Sigma-Aldrich, 1:400). Immunoreactions were visualized by donkey anti-rabbit Alexa 594 (Molecular Probes), and observed by a fluorescent microscope (Carl Zeiss). Serum shock analysis of BSMC Primary BSMC, isolated from female SD rats aged 9 weeks [22] , [56] , were cultured after two passages until sub-confluent in DMEM with 10% FCS and 1% penicillin streptomycin followed by 72 h incubation in DMEM with 0.5% FCS. The cells were treated with 50% horse serum (GIBCO-BRL) in DMEM for 2 h (ref. 39 ), and washed twice with DMEM, and then maintained in DMEM with 0.5% FCS for a maximum of 72 h. Immunostaining of BSMC BSMC were serum-shocked and fixed with 4% formaldehyde, permeabilized with 0.4% Triton X-100, and blocked with 10% goat serum (Invitrogen). The cells were incubated with Cx43 rabbit polyclonal antibody (Sigma-Aldrich, 1:500) followed by goat anti-rabbit Alexa 594 (Molecular Probes) and counter stained with 4,6-diamidino-2-phenylindole (DAPI) [57] . Lucifer yellow microinjections Nuclei of serum-shocked BSMC were pre-stained with 16 μM of Hoechst 33342 (Invitrogen) for 15 min, to identify the site of injection. A single cell was impaled with a microelectrode, and Lucifer Yellow was injected by an electrometer (model 3100; A-M systems) for 1 min with a continuous current of 0.1 μA. Images were acquired using a CoolSNAP-HQ2 CCD camera (Photometrics) [57] . Fluorescent cells were counted and the values were normalized by the total number of cells within the injected region of interest, with a mean cell density of 32.6±6.6 cells). Promoter-reporter assay The promoter–reporter constructs used were, mouse pGL-2-Cx43 (pCx43 −1686/+165-luc) 42 , mouse pGL-3-Per1 (pPer1-luc), pGL-3-Bmal1 (pBmal1-luc), and pGL-2 basic, pRL-TK (Promega) as controls. The expression vectors used were, Sp1 and Sp3 (fully lengthened according to a previous report) [58] , [59] , Clock, Bmal1, Cry1, Dbp, E4bp4, Rev-erbα and Rorα (Open Biosystems). Site-directed mutagenesis, deletion and addition of aimed sequences were performed using a mutagenesis basal kit (Takara). Corrected mutants were all verified by sequencing. For luciferase assays, reporter plasmids (100 ng) with various expression vectors (total 250 ng) were transfected to HEK293T cells in 24-well plates and those (total 100 ng) to BSMC in 96-well plates using Fugene6 (Roche) in DMEM with 10% FCS. Plasmid dosage was kept constant by the EGFP-N1 vector. Lysates were collected 48 h post-transfection, and the luciferase activity was measured using a dual luciferase assay reagent (Promega). RNA interference assay Three sets of Stealth Select RNAi targeted against rat Rev-erbα (Rat Nr1d1 1330003) and Stealth RNAi Negative Control (low, medium and high GC, Invitrogen) were used. After two passages, BSMC were plated on 6-well plates and kept for 24 h in DMEM with 10% FCS. This was followed by transfection of siRNA (75 pmol per well) in serum-reduced αMEM for 5 h using Lipofectamin RNAiMAX (Invitrogen), followed by medium-change to DMEM with 10% FCS. After 48 h of the transfection, total RNA and cell lysates were extracted. Co-immunoprecipitation assay Rev-erbα with amino-terminal MYPYDVPDYA-tag (HA-Rev-erbα) and Sp1 with N-terminal MDYKDDDDK-tag (DDDDK-Sp1) were constructed using a mutagenesis basal kit (Takara). Nuclear extracts were prepared from HEK293T cells transfected with expression vectors for 48 h, using a Nuclear Complex Co-IP kit (Active Motif). A total of 100 μg of nuclear extracts were incubated with antibodies for 0.27 μg of Rev-erbα (Cell Signalling), 4 μg of HA (Abcam), DDDDK (MBL) and control rabbit IgG (Zymed), in 500 μl of low IP buffer overnight at 4 °C with rotation followed by the addition of 30 μl of Dynabeads Sheep anti-Rabbit IgG (Veritas) for 1 h. After washing with low IP buffer with/without BSA three times each, the binding protein was eluted in 40 μl of radioimmunoprecipitation assay buffer for immunoblotting. A total of 2 μg of nuclear extracts were used as input. Chromatin immunoprecipitation Formaldehyde-crosslinked chromatins were obtained from HEK293T cells and serum-shocked BSMC, which were sheared using Chip-IT Express Enzymatic (Active Motif). Sheared chromatins were immunoprecipitated with antibodies to 0.23 μg of Rev-erbα (Lifespan Biosciences, LS-C37817), 2 μg of HA, DDDDK and control rabbit IgG overnight at 4 °C with rotation followed by the addition of 15 μl of Dynabeads Sheep anti-Rabbit IgG for 1 h. The Chip-IT control kits Rat and Human (Active Motif) were used as an experimental control. The enrichment of Sp1-binding sequences in eluted DNA was de-crosslinked by incubation at 65 °C, for 4 h, followed by digestion of protein by proteinase K. Purified DNA, using a QIAquick PCR purification kit (Qiagen), was quantified by real-time RT–PCR and normalized by the quantity of input DNA [60] . Samples of BSMC after real-time RT–PCR were visualized by electrophoresis. Primers used are listed in Supplementary Table S1 . Microarray analysis of the mouse bladder Whole bladder RNA of female C57BL/6 mice killed at CT 0, 4, 8, 12, 16 and 20 as described above was used ( n =2 for each time point). A total of 250 ng of qualified RNA was employed for the synthesis of Cy3-labelled antisense RNA, which was qualified and hybridized to the Whole Mouse Genome Oligo Microarray (44K; Agilent Technologies) according to the manufacturer's protocol (entrusted to DNA Chip Research, Yokohama, Japan). Statistical analysis of microarray data was performed using R statistical software (version 2.8.1, 2008-12-22) with BioConductor (version 2.3). Signal processing was performed by Agilent Feature Extraction (version. 9.5.3). Normalization was performed based on the Agi4x44PreProcess package (version 1.2.0). The mgug4122a.db package (version 2.2.5) was used for annotation of each probe. Selection of circadian-oscillated genes was based on the modified procedure of Yamada et al . [35] and McDonald et al . [34] . Specifically, we calculated correlation coefficients between each six-point time course and 60 different-phased cosine curves with six time points. For each probe, we selected one cosine curve with MaxCorr from the 60 different-phased cosine curves. The false-positive proportion was estimated on the basis of the null distribution of maximum correlations derived from randomly generated expression profiles. Statistical analysis For the micturition experiments, we used one-way ANOVA with Bonferroni's post hoc test to evaluate differences among time points. Two-way repeated measures ANOVA was used to compare differences between the two groups of mice tested, and time points were compared with Bonferroni's post hoc test. For the experiments in which three or more test groups were compared, we used one-way ANOVA, and for those including two factors, we used two-way ANOVA. Accession codes: Microarray data have been deposited in the Gene Expression Omnibus under accession code GSE35795 . How to cite this article: Negoro, H. et al . Involvement of urinary bladder Connexin43 and the circadian clock in coordination of diurnal micturition rhythm. Nat. Commun. 3:809 doi: 10.1038/ncomms1812 (2012).